Integrated control of hepatic lipogenesis versus glucose production requires FoxO transcription factors Insulin integrates hepatic glucose and lipid metabolism, directing nutrients to storage as glycogen and triglyceride. In type 2 diabetes, levels of the former are low and the latter are exaggerated, posing a pathophysiologic and therapeutic conundrum. A branching model of insulin signalling, with FoxO1 presiding over glucose production and Srebp-1c regulating lipogenesis, provides a potential explanation. Here we illustrate an alternative mechanism that integrates glucose production and lipogenesis under the unifying control of FoxO. Liver-specific ablation of three FoxOs (L–FoxO1,3,4) prevents the induction of glucose-6-phosphatase and the repression of glucokinase during fasting, thus increasing lipogenesis at the expense of glucose production. We document a similar pattern in the early phases of diet-induced insulin resistance, and propose that FoxOs are required to enable the liver to direct nutritionally derived carbons to glucose versus lipid metabolism. Our data underscore the heterogeneity of hepatic insulin resistance during progression from the metabolic syndrome to overt diabetes, and the conceptual challenge of designing therapies that curtail glucose production without promoting hepatic lipid accumulation. The integrative regulation of hepatic carbohydrate and lipid metabolism by insulin is a key biological question with important ramifications for the pathogenesis and potential treatment of type 2 diabetes [1] . Diabetics overproduce glucose and triglycerides, contributing to the twin abnormalities of this disease, hyperglycaemia and hypertriglyceridemia [2] . Less clear is how these actions of insulin are mediated, and why they are inextricably linked in the pathogenesis of insulin resistance, the forerunner of type 2 diabetes Insulin’s repression of hepatic glucose production (HGP) [2] is mediated by the Irs–Akt–FoxO pathway [3] , [4] , [5] , [6] , [7] . Conversely, insulin promotes de novo lipogenesis (DNL), through Akt-mediated activation of Srebp-1c [8] , [9] , [10] . A widely held model suggests that insulin signalling bifurcates downstream of Akt, to regulate HGP and DNL separately, through these two independent, parallel effectors [1] . In contrast to this model, evidence suggests that FoxOs are also required for normal regulation of lipid synthesis and metabolism [6] , [11] , [12] , [13] , [14] , [15] , [16] . FoxOs are thought to promote HGP primarily by activating transcription of glucose-6-phosphatase (encoded by G6pc ) [2] . However, there are two problems with this explanation: first, G6pc enzyme levels are at best modestly correlated with HGP in diabetes [17] , and second, the effect of liver FoxO ablation on HGP vastly exceeds its effect on G6pc [3] , [5] , [7] . Moreover, mice with a triple knockout of Akt1/Akt2/FoxO1 in the liver (or Irs1/Irs2/FoxO1) have a transcriptional response to fasting and refeeding (F–RF) that is similar to controls [4] , [5] , raising the question of whether and how FoxOs are required for the F–RF response. We expected that a major reason for the mild defects observed after FoxO1 knockout is the redundancy of FoxOs [3] , [5] . We employed a combination of genetic, metabolomic and flux analysis in L–FoxO1,3,4 mice to address two goals: (i) to critically test the model that FoxOs promote HGP but do not regulate DNL and (ii) to examine the requirement for FoxOs during the F–RF transition in healthy mice. We report that FoxOs exert dual control over G6pc and glucokinase ( Gck ), thus determining whether glucose-6-phosphate is routed towards glucose versus lipid metabolism. Hepatic FoxOs control the G6pc/Gck ratio We found that 30% of L–FoxO1,3,4 mice die before weaning ( Fig. 1a ), possibly because of fatal postnatal hypoglycaemia ( Supplementary Fig. 1a ) [7] . Surviving adult L–FoxO1,3,4 mice presumably have the most robust compensatory mechanisms but still showed low glucose and insulin during daytime ad libitum feeding, and hypoglycaemia after prolonged fasting ( Supplementary Fig. 1b–c ) [7] , [18] . In hyperinsulinemic–euglycaemic clamps, L–FoxO1,3,4 mice required double the glucose infusion rate of controls ( Fig. 1b ). There was no significant difference in glucose disposal; however, L–FoxO1,3,4 mice showed ~60% reduction in HGP ( Fig. 1c,d ). 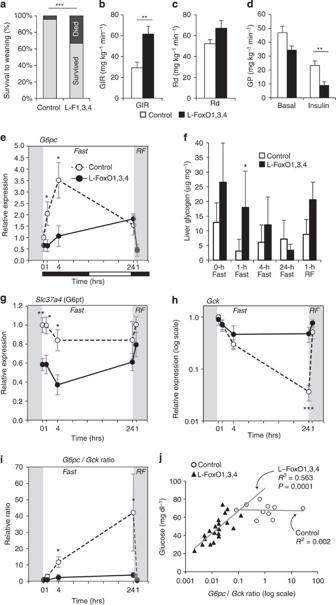Figure 1: Glucose parameters in L–FoxO1,3,4 mice. (a) Percentage of pups surviving to weaning at 21 days.n=70 control and 24 L–FoxO1,3,4 pups. ***P<0.001 by Fisher’s exact test. These numbers may underestimate the true mortality of L–FoxO1,3,4 pups; at genotyping (day 9) they are already present at less than Mendelian ratios7. (b–d) During hyperinsulinemic–euglycaemic clamp (n=8 controls, 6 L–FoxO1,3,4): (b) glucose infusion rate (GIR); (c) rate of glucose disposal (Rd); (d) glucose production (GP) **P<0.01 by Student’st-test (two-tailed). (e–i) Liver gene expression and glycogen content during F-RF time course (n=4–7, exactnfor each time point and genotype listed in Methods): (e)G6pcexpression; (f) liver glycogen; (g)Slc37a4, encoding the glucose-6-phosphate transporter; (h)Gck; (i)G6pc/Gckratio. ***P<0.001, **P<0.01, *P<0.05 for control versus L–FoxO1,3,4 mice by Student’st-test (two-tailed). Black and white bars indicate the dark/light cycle. (j) Correlation between glucose levels and theG6pc/Gckratio in pups at P2. Data are mean±s.e.m. Figure 1: Glucose parameters in L–FoxO1,3,4 mice. ( a ) Percentage of pups surviving to weaning at 21 days. n =70 control and 24 L–FoxO1,3,4 pups. *** P <0.001 by Fisher’s exact test. These numbers may underestimate the true mortality of L–FoxO1,3,4 pups; at genotyping (day 9) they are already present at less than Mendelian ratios [7] . ( b – d ) During hyperinsulinemic–euglycaemic clamp ( n =8 controls, 6 L–FoxO1,3,4): ( b ) glucose infusion rate (GIR); ( c ) rate of glucose disposal (Rd); ( d ) glucose production (GP) ** P <0.01 by Student’s t -test (two-tailed). ( e – i ) Liver gene expression and glycogen content during F-RF time course ( n =4–7, exact n for each time point and genotype listed in Methods): ( e ) G6pc expression; ( f ) liver glycogen; ( g ) Slc37a4 , encoding the glucose-6-phosphate transporter; ( h ) Gck ; ( i ) G6pc / Gck ratio. *** P <0.001, ** P <0.01, * P <0.05 for control versus L–FoxO1,3,4 mice by Student’s t -test (two-tailed). Black and white bars indicate the dark/light cycle. ( j ) Correlation between glucose levels and the G6pc / Gck ratio in pups at P2. Data are mean±s.e.m. Full size image We investigated transcriptional mechanisms of metabolic control by FoxO during fasting and refeeding (F–RF). In controls, G6pc peaked at 4 h of fasting; however, L–FoxO1,3,4 mice were unable to induce this peak ( Fig. 1e ). Consistent with this, fasting L–FoxO1,3,4 mice showed delayed glycogen depletion ( Fig. 1f ). Igfbp1 —a canonical FoxO target—showed an expression pattern similar to G6pc ; however, there was no defect in the expression of Pck1 in L–FoxO1,3,4 mice ( Supplementary Fig. 1d–e ). We unexpectedly identified a 40% decrease in expression of the glucose-6-phosphate transporter ( Fig. 1g ). Thus, this transporter may contribute to FoxO’s control of glucose release from the liver [19] , although it was not strongly regulated by F–RF. Next, we measured expression of glucokinase (encoded by Gck ), which is critical for hepatic glucose utilization [20] , [21] , [22] , [23] , [24] , [25] , [26] , [27] , and is negatively regulated by FoxOs [7] , [15] , [18] , [28] . In controls, Gck was strongly suppressed during fasting and induced within 1 h of RF ( Fig. 1h ). In contrast, in L–FoxO1,3,4 mice, Gck was hardly suppressed during fasting. Notably, Gck expression in L–FoxO1,3,4 mice fasted for 24 h was similar to controls RF for 1 h, demonstrating that inactivating FoxOs mimics the early effect of refeeding on Gck . As G6pc opposes Gck to control the intracellular gradients of glucose and glucose-6-phosphate, the ratio of the two enzymes may reflect the direction of glucose flux. In control mice, the G6pc / Gck ratio was potently induced during fasting, consistent with increased hepatic glucose output; however, this effect was completely absent in L–FoxO1,3,4 mice ( Fig. 1i ). Furthermore, the ratio of G6pc / Gck was the strongest predictor of glycaemia in L–FoxO1,3,4 pups ( R =0.75; P =0.0001; Fig. 1j ). This was not true in control pups, which showed nearly undetectable Gck, as expected [29] , [30] , [31] . This suggests that G6pc is only rate-limiting in the presence of counteraction by Gck. Analysed individually, Gck was less strongly correlated to glucose, as was G6pc ( Supplementary Fig. 1f–g ). To buttress the conclusion that FoxOs are important for regulation of the transcriptional response F–RF, we performed unbiased surveys of expressed mRNAs. Analyses of global gene expression patterns after 22-h fasting or 4-h RF revealed that fasted L–FoxO1,3,4 mice largely resemble RF controls ( Supplementary Fig. 1h ). This demonstrated that inactivating FoxOs mimics the effect of RF on a large proportion of nutritionally regulated genes. Finally, we confirmed that FoxOs are required for induction of G6pc and suppression of Gck using primary hepatocytes derived from control or L–FoxO1,3,4 mice ( Supplementary Fig. 1i ). Glucose cycling and DNL in FoxO-deficient mice To investigate glucose uptake and utilization, we injected mice with a mixture of two stable isotope-labelled glucoses [32] . In control mice, both tracers peaked in blood 30 min after injection and were cleared within 2 h ( Fig. 2a,b ). At every time point, both tracers were reduced in L–FoxO1,3,4 mice ( Fig. 2a,b ), demonstrating increased glucose uptake and utilization. This can likely be attributed to the liver because glucokinase activators increase liver glucose uptake and glycolysis [33] , and because the rate of glucose disposal in the clamp (primarily reflecting glucose uptake in muscle and fat) showed no significant difference. Total plasma glucose and insulin were reduced in L–FoxO1,3,4, as expected [7] ( Supplementary Fig. 2a–c ). However, the fractional difference in enrichment of the two labels was the same in both genotypes ( Fig. 2c ), indicating no difference in the rate of glucose cycling [34] . 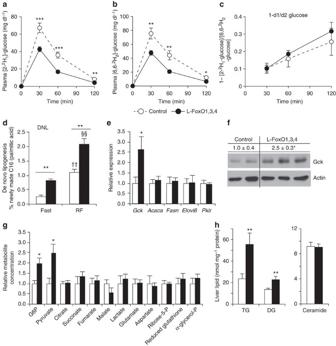Figure 2: Glucose utilization and lipogenesis. (a) Plasma levels of [2-2H1]-glucose after injection. (b) Plasma levels of [6,6-2H2]-glucose after injection. (c) Fractional difference in labelled glucose enrichment (n=9 control, 11 L–FoxO1,3,4). ***P<0.001, **P<0.01, *P<0.05 for control versus L–FoxO1,3,4 mice by Student’st-tests (two-tailed). (d)De novolipogenesis (n=4 control, fasted; 5 L–FoxO1,3,4, fasted; 7 control, RF; 5 L–FoxO1,3,4, RF). **P<0.01 for control versus L–FoxO1,3,4 mice;††P<0.01 for RF versus fasted control mice;§§P<0.01 for RF versus fasted L–FoxO1,3,4 mice by two-way analysis of variance. (e) Fasting gene expression (n=7 control; 5 L–FoxO1,3,4). *P<0.05. (f) Western blot of glucokinase in liver lysates from fasting mice (n=4 control; 5 L–FoxO1,3,4; representative blot shown). Numerical values above the blot are mean±s.e.m. of Gck/actin, relative to controls. *P<0.05. (g) Liver metabolites measured by GC–MS, relative to controls (n=4 control; 5 L–FoxO1,3,4). *P<0.05. (h) Liver lipidomic analyses. Total levels of the indicated lipid species. Full data set, including individual lipid species available inSupplementary Table 1(n=14 control; 11 L–FoxO1,3,4). **P<0.01 by Student’st-tests (two-tailed). Figure 2: Glucose utilization and lipogenesis. ( a ) Plasma levels of [2- 2 H 1 ]-glucose after injection. ( b ) Plasma levels of [6,6- 2 H 2 ]-glucose after injection. ( c ) Fractional difference in labelled glucose enrichment ( n =9 control, 11 L–FoxO1,3,4). *** P <0.001, ** P <0.01, * P <0.05 for control versus L–FoxO1,3,4 mice by Student’s t- tests (two-tailed). ( d ) De novo lipogenesis ( n =4 control, fasted; 5 L–FoxO1,3,4, fasted; 7 control, RF; 5 L–FoxO1,3,4, RF). ** P <0.01 for control versus L–FoxO1,3,4 mice; †† P <0.01 for RF versus fasted control mice; §§ P <0.01 for RF versus fasted L–FoxO1,3,4 mice by two-way analysis of variance. ( e ) Fasting gene expression ( n =7 control; 5 L–FoxO1,3,4). * P <0.05. ( f ) Western blot of glucokinase in liver lysates from fasting mice ( n =4 control; 5 L–FoxO1,3,4; representative blot shown). Numerical values above the blot are mean±s.e.m. of Gck/actin, relative to controls. * P <0.05. ( g ) Liver metabolites measured by GC–MS, relative to controls ( n =4 control; 5 L–FoxO1,3,4). * P <0.05. ( h ) Liver lipidomic analyses. Total levels of the indicated lipid species. Full data set, including individual lipid species available in Supplementary Table 1 ( n =14 control; 11 L–FoxO1,3,4). ** P <0.01 by Student’s t -tests (two-tailed). Full size image Increased Gck is expected to increase DNL [23] , [24] , [35] , and we next measured the rate of DNL during F–RF. In control mice, DNL was low after an 18-h fast and quadrupled after 5-h RF; however, L–FoxO1,3,4 mice showed two to three times higher rates of DNL at both time points ( Fig. 2d ). We noted that DNL in 18-h-fasted L–FoxO1,3,4 mice was nearly as high as in 5-h-refed controls, indicating that FoxO inactivation mimics the effect of 5-h refeeding on lipogenesis. We next investigated lipogenic pathways that could explain the increased DNL. During prolonged fasting (when L–FoxO1,3,4 mice have ~3 × higher DNL), we found no difference between genotypes in mRNA expression of target genes of canonical lipogenic transcription factors Srebp-1c and Chrebp, including Acaca , Fasn , Elovl6 and Pklr ( Fig. 2e ). Thus, increases in Srebp-1c or Chrebp function cannot explain the increased lipogenesis in L–FoxO1,3,4 mice, while increased Gck can ( Fig. 2e,f ). Metabolomic and lipidomic analyses revealed that L–FoxO1,3,4 livers had increased G6P, pyruvate, triglycerides, and diglycerides ( Fig. 2g,h , Supplementary Table 1 ), consistent with increased glycolysis and lipogenesis. Other metabolites showed no significant differences, except a trend towards reduced malate, potentially indicating that TCA cycle flux is preferentially re-routed into lipogenesis. The increased diglycerides were surprising, as they have been suggested to engender insulin resistance [36] , and L–FoxO1,3,4 mice are exceedingly insulin-sensitive. Our data suggest that derepression of Gck may be an exquisitely insulin-sensitive mechanism to activate DNL [23] , [24] , [35] independently of canonical lipogenic pathways. We examined this in more detail in C57BL/6J mice during F–RF. Both Elovl6 (Srebp-1c target) and Pklr (Chrebp target) were reduced during fasting and increased after refeeding, as expected ( Fig. 3a ). In contrast, the fluctuations of Gck were greater during F–RF, and peaked within 1 h of refeeding, hours before Srebp-1c and Chrebp targets. We confirmed that Gck protein was induced within 1 h of refeeding ( Supplementary Fig. 3a ). 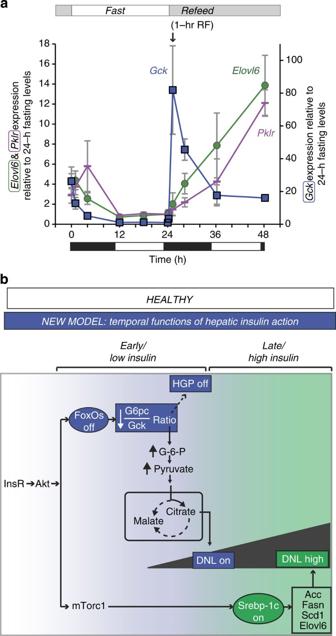Figure 3: Lipogenic gene expression during F–RF in chow-fed C57BL/6J mice and proposed physiologic model. (a) Comparison ofGck, Elovl6andPklrexpression. For each gene, the 24-h fasting time point is set equal to 1.Elovl6andPklrare plotted using the vertical axis on the left, andGckis plotted using the vertical axis on the right.n=5 per group. Black and white bars indicate the dark/light cycle. (b) Model. Earlier data suggested parallel action of insulin through FoxO to regulate HGP, and through Srebp-1c to regulate DNL. We propose a new model, whereby insulin acts first at low levels and early time points through FoxOs to reduce HGP and initiate postprandial DNL by reducing theG6pc/Gckratio, and second at high levels and late time points through Srebp-1c to amplify DNL. Figure 3: Lipogenic gene expression during F–RF in chow-fed C57BL/6J mice and proposed physiologic model. ( a ) Comparison of Gck, Elovl6 and Pklr expression. For each gene, the 24-h fasting time point is set equal to 1. Elovl6 and Pklr are plotted using the vertical axis on the left, and Gck is plotted using the vertical axis on the right. n =5 per group. Black and white bars indicate the dark/light cycle. ( b ) Model. Earlier data suggested parallel action of insulin through FoxO to regulate HGP, and through Srebp-1c to regulate DNL. We propose a new model, whereby insulin acts first at low levels and early time points through FoxOs to reduce HGP and initiate postprandial DNL by reducing the G6pc / Gck ratio, and second at high levels and late time points through Srebp-1c to amplify DNL. Full size image New model of insulin control of hepatic glucose versus lipid metabolism Our data demonstrate that FoxOs regulate both glucose and lipid production, and suggest a new model of the regulation of insulin of these two processes. Instead of parallel functions through FoxOs and Srebp-1c, we propose that insulin acts on them sequentially ( Fig. 3b ): first, hepatic FoxOs are inactivated, immediately inducing glucokinase. In combination with glucose-dependent dissociation of Gck from its regulatory protein, this amplifies lipogenesis. Second, the Srebp-1c pathway is activated, thereby enhancing DNL. Our model is supported by the fact that FoxOs are inactivated within seconds of exposure to physiologic (picomolar) insulin doses, whereas Srebp-1c activation requires hours and higher insulin doses [37] . This proposed model justifies detailed future investigation of the time course of postprandial induction of DNL. Moreover, it may be worth investigating whether dual effects of FoxOs on HGP and DNL are complementary to the effects of Hdac3 on hepatic metabolic routing [38] . To investigate the pathophysiologic implications of this model, we examined the effects of 1 week of western-type diet (WTD) feeding in C57BL/6J mice. This dietary challenge induced mild insulin resistance, as demonstrated by elevated glucose and insulin ( Fig. 4a,b ). This was associated with milder induction of G6pc and considerable blunting of Gck suppression during fasting ( Fig. 4c,d ). We confirmed that glucokinase protein was also increased in WTD-feeding ( Supplementary Fig. 3b ). Furthermore, WTD-fed mice showed marked decreases in the G6pc / Gck ratio during fasting ( Fig. 4e ). These data demonstrate that short-term WTD-feeding mimics FoxO loss-of-function. 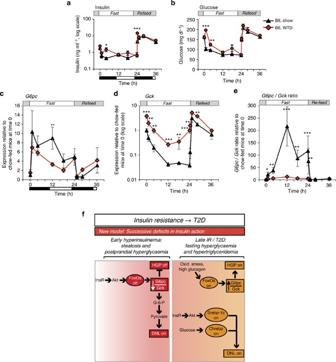Figure 4: Pathophysiology and model. (a) Insulin and (b) glucose during F–RF in C57BL/6J mice fed chow or WTD for 1 week.n=5 per group. (c)G6pcexpression, (d)Gckexpression and (e)G6pc/Gckratio from chow and WTD-fed C57BL/6J mice during F–RF. Expression in chow-fed mice at time 0 is set equal to 1.n=5 per group. Black and white bars indicate the dark/light cycle. *P<0.05; **P<0.01; ***P<0.001 for chow- versus WTD-fed mice by Student’st-tests (two-tailed). (f) Model of the progression of insulin resistance and type 2 diabetes. The current model suggests bifurcation of insulin signalling, such that the FoxO branch is resistant to insulin and the Srebp-1c branch is excessively activated by hyperinsulinemia. We propose a new model, with successive defects in hepatic insulin action. In early hyperinsulinemia, FoxOs are strongly suppressed, thereby decreasing theG6pc/Gckratio and activating lipogenesis. Later in disease progression, the Srebp-1c and Chrebp pathways are activated by insulin, whereas FoxOs may be activated by other mechanisms, for example, oxidative stress-induced acetylation or glucagon-induced alternative phosphorylation. Figure 4: Pathophysiology and model. ( a ) Insulin and ( b ) glucose during F–RF in C57BL/6J mice fed chow or WTD for 1 week. n =5 per group. ( c ) G6pc expression, ( d ) Gck expression and ( e ) G6pc / Gck ratio from chow and WTD-fed C57BL/6J mice during F–RF. Expression in chow-fed mice at time 0 is set equal to 1. n =5 per group. Black and white bars indicate the dark/light cycle. * P <0.05; ** P <0.01; *** P <0.001 for chow- versus WTD-fed mice by Student’s t -tests (two-tailed). ( f ) Model of the progression of insulin resistance and type 2 diabetes. The current model suggests bifurcation of insulin signalling, such that the FoxO branch is resistant to insulin and the Srebp-1c branch is excessively activated by hyperinsulinemia. We propose a new model, with successive defects in hepatic insulin action. In early hyperinsulinemia, FoxOs are strongly suppressed, thereby decreasing the G6pc / Gck ratio and activating lipogenesis. Later in disease progression, the Srebp-1c and Chrebp pathways are activated by insulin, whereas FoxOs may be activated by other mechanisms, for example, oxidative stress-induced acetylation or glucagon-induced alternative phosphorylation. Full size image The key novel conclusions of this work are as follows: (i) FoxOs are required for the dynamic regulation of G6pc / Gck during F–RF; (ii) this reciprocal regulation is a critical step in controlling hepatic glucose output and DNL; and (iii) short-term WTD-feeding induces a phenotype resembling liver FoxO inactivation. Data presented in this study suggest a new model of glucose and lipid dysregulation in the pathophysiology of insulin resistance, based on successive defects in insulin action ( Fig. 4f ): in mild/early insulin resistance, portal hyperinsulinemia drives FoxO inactivation. This leads to a decrease in the G6pc / Gck ratio and excess DNL at the expense of hepatic glucose output. As the disease advances, there is a further rise in insulin and glucose levels, leading to induction of Srebp-1c/Chrebp-dependent lipogenesis. In this severe disease setting, FoxOs can be reactivated through oxidative stress [39] , [40] or an adverse kinase profile favouring their nuclear retention [41] . This model, while partly still speculative, reconciles our molecular understanding of hepatic insulin signalling with the known clinical features of diabetes progression. Thus, in the early phases of the disease, hyperglycaemia is mostly postprandial, but liver steatosis is already present [42] . In the advanced disease, fasting hyperglycaemia accounts for a growing fraction of total glycaemic variation [43] . In this setting, the combination of active transcription factors heralds the increase in both HGP and lipogenesis that is typical of the diabetic state. Our data also help to reinterpret studies showing that hepatic insulin signalling occurs normally in the absence of Akt1/Akt2/FoxO1 (ref. 5 ) or Irs1/Irs2/FoxO1 (ref. 4 ). We show that the gene expression profile of fasted mice lacking the three FoxOs is strikingly similar to that of fed wild-type controls. This, in addition to the early postnatal death of a fraction of triple knockouts, and the profound flux abnormalities described in the survivors, should disabuse us of the notion that the FoxOs can be done away with. First, we suggest that the combined knockouts of Akt or Irs with FoxO1 did not account for the functions of FoxO3a and 4, which we show to be substantial. Second, the ability of insulin to suppress HGP in clamp studies of Akt1/Akt2/FoxO1 mutants, which we confirm in triple FoxO knockouts in the present study, likely reflects two things: (1) the extrahepatic actions of insulin, for example, through free fatty acids (FFAs) or the central nervous system (CNS) [2] and (2) the contrived conditions of the clamp, wherein insulin levels are raised many fold over the physiologic range. The novel models of insulin–FoxO regulation of HGP and DNL in normal physiology ( Fig. 3b ) and in the pathophysiology of diabetes ( Fig. 4f ) underscore the conceptual advances arising from this work. These findings should prompt a reappraisal of the heterogeneity of hepatic insulin resistance during the transition from the metabolic syndrome to overt diabetes. They also provide a powerful illustration of the conceptual and regulatory challenges underlying the development of new treatments for this condition. Mice and diets L–FoxO1,3,4 mice have been described [7] . Only males at least 16 weeks old were studied, except in studies of 2-day-old pups, where pups of both genders were used. Male C57BL/6J mice were purchased from Jackson Laboratory and were studied when they were 9 weeks old. All mice were fed chow, except in the experiment shown in Fig. 4a–e , where C57BL/6J mice were challenged with WTD for 1 week. WTD is from Harlan Teklad (TD.88137); it contains ~30% kcal from sucrose and 42% from fat, and causes insulin resistance. [12] Mice were maintained on a 12-h light–dark cycle (lights on at 0700 hours). The Columbia University Institutional Animal Care and Utilization Committee approved all experiments. Metabolic tests Blood glucose was measured using OneTouch glucose monitor and strips (Lifescan). Insulin ELISAs were from Millipore. Hyperinsulinemic–euglycaemic clamps were carried 5–6 h after removing food. We infused a solution of glucose (10%) at a variable rate to maintain plasma glucose ~8 mM. Mice received a constant infusion of [3- 3 H] glucose (0.1 mCi min −1 ) and insulin (3.6 mU per kg body weight per min). We collected plasma samples to determine glucose levels at times 10, 20, 30, 40, 50, 60, 70, 80 and 90 min after beginning insulin and glucose infusions, and measured the specific activities of [3- 3 H] glucose and 3 H water at 40, 50, 60, 70, 80 and 90 min after beginning the insulin and glucose infusions. We achieved steady-state conditions for plasma glucose concentration and specific activity within 40 min from the beginning of the insulin clamp. During the last 10 min of the clamp study, we infused a solution of [U- 14 C] lactate in normal saline (5 μCi as initial bolus, followed by 0.25 μCi min −1 ). At the end of the in vivo studies, mice were anaesthetised, their abdomens were quickly opened, portal blood was collected and livers were freeze-clamped in situ and stored at –80 °C for further analysis [44] . Hepatic recycling glucose tolerance tests (HR–GTTs) were carried out using a mixture of [2- 2 H] glucose (0.5 mg per g body weight) and [6,6- 2 H 2 ] glucose (0.5 mg g −1 ). When [2- 2 H]- and [6,6- 2 H 2 ] glucose are administered as a 1:1 mixture, the disappearance of the two isotopes [2- 2 H]- and [6,6- 2 H 2 ] glucose can be determined with mass fragmentography. The difference between the two disappearance rates is used to measure futile cycling. During the HR–dGTT, hepatic uptake of [2- 2 H] glucose generally leads to the loss of deuterium label at the C2 position because of isomerization between glucose-6-P and fructose-6-phosphate [32] . To measure DNL [45] , following IP injection of deuterated saline, drinking water was replaced with 6% D 2 O. Following a 1-h equilibration period, mice were either refed chow and killed 5 h later, or remained fasting for 18 h. Newly synthesized palmitate was measured using GC–MS [46] . For time course studies in control versus L–FoxO1,3,4, mice (shown in Fig. 1e–i ), mice were first synchronized by removing food during daytime (10:00–17:00 hours), and then food was replaced at 17:00 hours. The experimental fasting period began at 19:00 hours. Mice were killed at time 0 ( n =5 control; 5 L–FoxO1,3,4); 1-h fast ( n =6 control; 5 L–FoxO1,3,4); 4 h fast ( n =6 control; 4 L–FoxO1,3,4); 24 h fast ( n =6 control, 4 L–FoxO1,3,4); and 1 h refed ( n =6 control, 4 L–FoxO1,3,4). For time course studies in C57BL/6J mice (shown in Figs 3a and 4a–e ), the experiment was performed the same way, except the experimental fasting period began at 20:00 hours. Glycogen measurement Tissue was homogenized in 6% perchloric acid and centrifuged at 13,000 × g for 10 min at 4 °C. The supernatant was combined with an equal volume of distilled water and centrifuged at 13,000 × g for 10 min at 4 °C. The supernatant was neutralized to pH 7 with KOH, centrifuged at 13,000 × g for 10 min at 4 °C and the supernatant was incubated with amyloglucosidase at 42 °C for 2 h. Released glucose was quantified using a glucose assay kit (Sigma, GAHK20). mRNA and protein expression Liver RNA was prepared using Trizol, cDNA was synthesized using qScript (Quanta), and quantitative PCR was performed using goTaq (Promega). Primer sequences are available in Supplementary Table 2 . Western blots used the primary antibodies directed against the following proteins: Gck (a kind gift from Mark Magnuson) was used at a 1:1,000 dilution and actin (Abgent no. AM1829b) was used at 1:5,000. Western were quantitated using Image J. Metabolomics Liver tissue samples from fasted/refed experiments were extracted in ice-cold methanol/water (1:1) [46] . The relative concentrations of each metabolite were calculated using the area under the peak of M0 (unlabelled target ion) normalized to the internal standard and tissue weight. Lipidomics Liver tissue samples were collected after 5-h daytime fast. Lipid analysis was performed with liquid chromatography, electrospray ionization-tandem mass spectrometry (LC ESI-MS/MS) [47] . Microarray analyses We used GeneChip Mouse Exon arrays (Affymetrix) and the Partek Genomics Suite software. For heat map analysis, we used the criteria of false discovery rate <0.1, n =3 per group. Primary hepatocytes Isolated primary hepatocytes were plated in Medium 199+10% fetal bovine serum. Cells were serum-starved overnight in Medium 199+1% bovine serum albumin. After overnight starvation, appropriate cells were pretreated with 100 nM insulin for 1 h. Then, all cells were changed into serum-free medium containing (i) water+vehicle (EtOH); (ii) 0.1 M CPT-cAMP+1 μM dexamethasone; or (iii) cAMP/dex+100 nM insulin. Cells were incubated for 6 h in the treatment media and then harvested. Statistics and general methods Sample sizes were estimated from expected effect size based on previous experiments. No randomization was used. One mouse was excluded from analysis in the DNL experiment, as it had an unclear genotype. Four mice were excluded from the HR–GTT analysis because of problems detecting plasma enrichment of the stable isotope, suggesting a problem with the injection. One mouse was excluded from lipidomics analysis because of low levels of all lipid species. Most experiments were not blinded, with the exception of plasma glucose in P2 pups ( Fig. 1j ), as the pups were not genotyped at the time the glucose was measured. We utilized Student’s t -tests, two-way analysis of variance and Fisher’s exact tests, as appropriate. P values below 0.05 were considered significant. Accession codes: Microarray data have been deposited in Gene Expression Omnibus under accession code GSE60527 . How to cite this article: Haeusler, R. A. et al. Integrated control of hepatic lipogenesis versus glucose production requires FoxO transcription factors. Nat. Commun. 5:5190 doi: 10.1038/ncomms6190 (2014).